Novel sialic acid derivatives lock open the 150-loop of an influenza A virus group-1 sialidase Influenza virus sialidase has an essential role in the virus' life cycle. Two distinct groups of influenza A virus sialidases have been established, that differ in the flexibility of the '150-loop', providing a more open active site in the apo form of the group-1 compared to group-2 enzymes. In this study we show, through a multidisciplinary approach, that novel sialic acid-based derivatives can exploit this structural difference and selectively inhibit the activity of group-1 sialidases. We also demonstrate that group-1 sialidases from drug-resistant mutant influenza viruses are sensitive to these designed compounds. Moreover, we have determined, by protein X-ray crystallography, that these inhibitors lock open the group-1 sialidase flexible 150-loop, in agreement with our molecular modelling prediction. This is the first direct proof that compounds may be developed to selectively target the pandemic A/H1N1, avian A/H5N1 and other group-1 sialidase-containing viruses, based on an open 150-loop conformation of the enzyme. Influenza remains a serious health concern to humanity, with high morbidity and mortality rates [1] , [2] and the recent influenza A/H1N1 pandemic underscores the potential threat of this highly adaptive virus [3] . The sialidase (neuraminidase) of influenza virus has a major role in the virus' life cycle by facilitating release of virus progeny from the infected cell [4] . Two phylogenetically distinct groups [5] of influenza A virus sialidases, group-1 (N1, 4, 5 and 8) and group-2 (N2, 3, 6, 7 and 9), have been established. The anti-influenza drugs [6] ( Fig. 1 ) Relenza (zanamivir, 1 ) and Tamiflu (oseltamivir, 2 ), through its active form oseltamivir carboxylate (OC, 3 ), efficiently block the activity of both influenza A virus group-1 and group-2 sialidases, resulting in the virus progeny remaining clumped at the infected cell's surface. Noteworthy is that the discovery of these inhibitors was based exclusively on group-2 sialidase structures [6] . 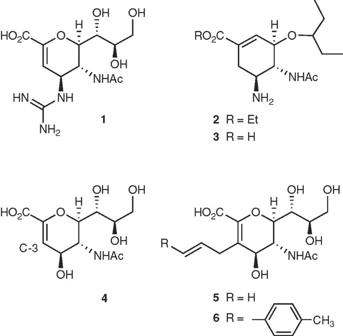Figure 1: Chemical structures of anti-influenza viral drugs and influenza virus sialidase inhibitors. Zanamivir (1), oseltamivir (2), oseltamivir carboxylate (3), Neu5Ac2en (4), 3-allyl-Neu5Ac2en (5) and 3-(p-tolyl)allyl-Neu5Ac2en (6). Figure 1: Chemical structures of anti-influenza viral drugs and influenza virus sialidase inhibitors. Zanamivir ( 1 ), oseltamivir ( 2 ), oseltamivir carboxylate ( 3 ), Neu5Ac2en ( 4 ), 3-allyl-Neu5Ac2en ( 5 ) and 3-( p -tolyl)allyl-Neu5Ac2en ( 6 ). Full size image The recently solved [5] structures of group-1 sialidases showed an unexpected structural difference between group-1 and group-2 sialidases, with the group-1 sialidases having a loop, the so-called '150-loop', that is flexible compared with the identical loop of the group-2 sialidases. This protein loop can provide either a more open (group-1) or closed (group-2) active site architecture in the apo form of the enzyme. Furthermore, the 150-loop, in initially complexed structures of 3 –group-1 sialidase [5] , has been observed in the more open orientation and eventually closes and tightly coordinates 3 . In contrast, a very recent structural investigation on the 2009 pandemic H1N1 sialidase concluded that this group-1 enzyme seems to lack a 150-cavity [7] . It has been proposed that the more open enzyme architecture and consequently larger active site cavity in the apo structures of the group-1 sialidases could provide new opportunities for inhibitor design [5] , [6] , [8] , [9] . In the context of the recent pandemic swine origin A/H1N1 and the pandemic 1918 A/H1N1 influenza viruses, as well as the continuing threat of avian A/H5N1, such inhibitors could lead to new anti-influenza drugs that would add to the very limited number of treatment options available. The potent influenza virus sialidase inhibitors 1 and 3 show essentially comparable inhibition of influenza A virus group-1 and 2 sialidases [8] . This is not surprising as these inhibitors do not have the capacity to maintain the 150-loop of group-1 sialidases in an open orientation. An important question remains to be answered—could the 150-loop of influenza A virus group-1 sialidases be locked open to provide new opportunities in influenza virus sialidase inhibitor design? Moreover, could such 'designer' compounds that lock open this loop also selectively inhibit group-1 sialidases, including the pandemic swine origin H1N1 sialidase. Interestingly, C-4-modified zanamivir ( 1 ) derivatives have been recently reported that are believed to take advantage of this open 150-loop feature, although neither selectivity nor structural data have been presented in support of this conclusion [10] . More recently OC ( 3 ) analogues have been reported [11] that efficiently inhibit and are selective for a group-1 influenza virus sialidase. These compounds are thought to access the 150-cavity, and preliminary nuclear magnetic resonance (NMR) spectroscopic evidence for this conclusion is reported. To probe and attempt to lock open the 150-loop of influenza virus group-1 sialidases, we have undertaken a multidisciplinary study that used molecular modelling, chemical synthesis, enzyme and cell-based assays and protein X-ray crystallography. We have successfully designed and synthesized novel C-3-substituted sialic acid-based derivatives that efficiently and selectively inhibit group-1 sialidase activity by locking open the flexible 150-loop. These derivatives contain the zanamivir ( 1 ) core structure, although they lack the C-4 guanidino moiety, and incorporate a hydrophobic entity at the C-3 position. Moreover, we have demonstrated that these inhibitors are also effective against influenza virus clinical isolates containing mutations in the sialidase glycoprotein that convey resistance to oseltamivir ( 2 ) and reduced sensitivity to zanamivir ( 1 ). Molecular modelling study of a group-1 sialidase Our modelling study commenced with the superimposition of two group-1 sialidase N8 structures, apo N8 (2ht5) and the N8– 4 complex (2htr), which contain an open and closed 150-loop, respectively. This provided an opportunity to view the well-known sialidase inhibitor 5-acetamido-2,6-anhydro-3,5-dideoxy- d - glycero - d - galacto -non-2-enonic acid (Neu5Ac2en, 4 , Fig. 1 ) modelled in the context of a sialidase active site with an open 150-loop conformation. We concluded from this inspection that carbon-3 (C-3) of Neu5Ac2en ( 4 ) is oriented towards the 150-cavity in the more open form of the enzyme. As a consequence, we then used 4 as a template (Methods) to design probes of this cavity. This design study suggested that 4 modified at C-3 should be able to bind to the active site of apo -N8 with minimal distortion of the normal binding mode. Moreover, our modelling indicated that hydrophobic functionalities, such as an allyl or arylallyl group, introduced at C-3 on template 4 , should be accommodated in the 150-cavity. Finally, our modelling study also suggested that such functionalities would lock open the 150-loop and, as a direct outcome, should be selective for the influenza A virus group-1 sialidases. Interestingly, the C-3 position on 4 , to the best of our knowledge, has never been functionalized. Synthesis of novel sialic acid derivatives To explore novel functionalization of the C-3 position of 4 , we chose chemistries that would introduce a functional group that could be readily elaborated. We believed that introduction of an allyl group would provide significant opportunity to elaborate the new functionality through olefin cross-metathesis reactions [12] . Our strategy to access this novel class of chemical probe utilized the per- O -acetylated, methyl ester derivative of 4 ( Fig. 2 , Supplementary Methods ). From this derivative, we were able to readily prepare the target compounds ( Fig. 1 ), 3-allyl-Neu5Ac2en ( 5 ) and 3-( p -tolyl)allyl-Neu5Ac2en ( 6 ). 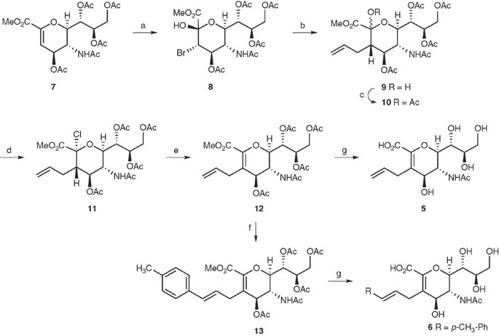Figure 2: Preparation of 3-allyl-Neu5Ac2en (5) and 3-(p-tolyl)allyl-Neu5Ac2en (6). Reagents and conditions: (a) NBS, DMSO/H2O (2.5:1), −30 °C, 2 h (38% di-equatorial bromohydrin8, 28% di-axial bromohydrin); (b) Bu3SnAll, AIBN, dry toluene, N2, 100 °C, 8 h (57%); (c) Ac2O, dry pyridine, DMAP, N2, room temperature, 16 h (95%); (d) AcCl, dry MeOH, dry DCM, 5 °C to room temperature, 48 h; (e) DBU, dry DCM, N2, room temperature, 8 h (91% over steps d and e, based on recovered starting material); (f) Grubbs' catalyst second generation, 4-methylstyrene, dry DCM, N2, 40 °C, 24 h (69%; 77% based on recovered starting material). (g) 1 M aq. NaOH, MeOH, 5 °C to room temperature, 12–16 h (5and6, 60%, based on recovered starting material, and 94%, respectively). Figure 2: Preparation of 3-allyl-Neu5Ac2en ( 5 ) and 3-( p -tolyl)allyl-Neu5Ac2en ( 6 ). Reagents and conditions: ( a ) NBS, DMSO/H 2 O (2.5:1), −30 °C, 2 h (38% di-equatorial bromohydrin 8 , 28% di-axial bromohydrin); ( b ) Bu 3 SnAll, AIBN, dry toluene, N 2 , 100 °C, 8 h (57%); ( c ) Ac 2 O, dry pyridine, DMAP, N 2 , room temperature, 16 h (95%); ( d ) AcCl, dry MeOH, dry DCM, 5 °C to room temperature, 48 h; ( e ) DBU, dry DCM, N 2 , room temperature, 8 h (91% over steps d and e, based on recovered starting material); ( f ) Grubbs' catalyst second generation, 4-methylstyrene, dry DCM, N 2 , 40 °C, 24 h (69%; 77% based on recovered starting material). ( g ) 1 M aq. NaOH, MeOH, 5 °C to room temperature, 12–16 h ( 5 and 6 , 60%, based on recovered starting material, and 94%, respectively). Full size image Biological evaluation of sialic acid derivatives To assess the ability of these compounds to selectively block the enzyme activity of group-1 influenza A virus sialidases, 5 and 6 have been evaluated in an in vitro fluorometric assay [13] against both wild-type and mutant group-1 (N1) and a wild-type group-2 (N2) viral sialidase (Methods). As anticipated, both probes 5 and 6 indeed showed selectivity for the group-1 (N1) sialidases compared with the group-2 (N2) sialidase ( Table 1 ), with a micromolar level of inhibition determined for 6 against the N1 sialidases. This is in distinct contrast to the parent inhibitor Neu5Ac2en ( 4 ), also a micromolar inhibitor, that shows comparable inhibition of both group-1 and group-2 sialidases. These data support the notion that 5 and 6 access a novel subsite within the influenza virus group-1 sialidase active site, such as that observed in the open 150-loop conformation [5] . Moreover, both of the sialic acid-based probes displayed activity against N1 sialidases associated with clinically relevant viruses [8] with mutations that affect sensitivity to both 1 and 2 ( Table 1 ). Finally, the selectivity for inhibition of N1 over N2 sialidase activity, shown by 5 and 6 , was confirmed by plaque reduction assay studies ( Supplementary Fig. S1 ) and 50% effective concentration (EC 50 ) determinations ( Supplementary Table S1 ). Table 1 Selective inhibition of influenza A group-1 sialidase by locking open the 150-loop. Full size table Structures of group-1 sialidase N8–5 and 6 complexes Influenza virus sialidase N8 [A/duck/Ukraine/1/63 (H3N8)] was used as a convenient and representative group-1 sialidase for structural studies. Both probes 5 and 6 were successfully complexed with N8 and structures readily determined. Both inhibitors 5 and 6 in complex with N8 (N8– 5 , Fig. 3 , Supplementary Fig. S2 , Supplementary Movie 1 ; N8– 6 , Fig. 4 , Supplementary Fig. S3 , Supplementary Movie 2 ) clearly demonstrated that the C-3 functionalities occupied the cavity formed by the open 150-loop. 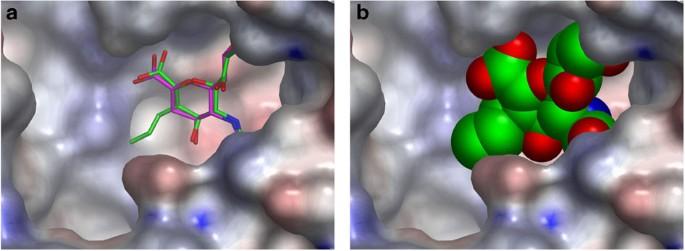Figure 3: N8–5complex. (a) Superimposition of N8–inhibitor complexes of 3-allyl-Neu5Ac2en (5, green) and Neu5Ac2en (4, magenta; 2htr). (b) N8–5complex with open 150-loop (5in CPK format). The N8–5complex maintains the open conformation of the 150-loop seen in theapostructure5(a, b). Figure 3: N8– 5 complex. ( a ) Superimposition of N8–inhibitor complexes of 3-allyl-Neu5Ac2en ( 5 , green) and Neu5Ac2en ( 4 , magenta; 2htr). ( b ) N8– 5 complex with open 150-loop ( 5 in CPK format). The N8– 5 complex maintains the open conformation of the 150-loop seen in the apo structure [5] (a, b). 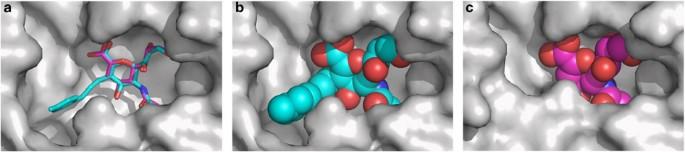Figure 4: N8–6 complex. (a) Superimposition of N8–inhibitor complexes of 3-(p-tolyl)allyl-Neu5Ac2en (6, cyan) and Neu5Ac2en (4, magenta; 2htr). (b) N8–6complex with an open 150-loop (6in CPK format). (c) N8–4complex with a closed 150-loop5(4in CPK format). The N8–6complex maintains an open conformation of the 150-loop seen in theapostructure5(a, b), in contrast to the complex with4where the 150-loop is closed (c). Full size image Figure 4: N8–6 complex. ( a ) Superimposition of N8–inhibitor complexes of 3-( p -tolyl)allyl-Neu5Ac2en ( 6 , cyan) and Neu5Ac2en ( 4 , magenta; 2htr). ( b ) N8– 6 complex with an open 150-loop ( 6 in CPK format). ( c ) N8– 4 complex with a closed 150-loop [5] ( 4 in CPK format). The N8– 6 complex maintains an open conformation of the 150-loop seen in the apo structure [5] (a, b), in contrast to the complex with 4 where the 150-loop is closed (c). Full size image On the basis of our structure-assisted studies, we identified 3-allyl-Neu5Ac2en ( 5 ) as an important versatile chemical intermediate for influenza virus sialidase inhibitor development. Our synthetic strategy to access 5 required the corresponding 3-substituted N -acetylneuraminic acid derivative, fully protected 3-allyl-Neu5Ac ( 10 ) ( Fig. 2 ). This derivative was synthesized from fully protected Neu5Ac2en ( 7 ) through bromohydroxylation [14] , and subsequent reaction of the di-equatorial bromohydrin 8 with allyltributyltin [15] . Reacting 8 with allyltributyltin in toluene at elevated temperature in the presence of the free radical initiator AIBN resulted in an improved yield of 9 (57%) compared with that reported [15] for the ultraviolet light-catalysed reaction (34%). Acetylation of 9 provided intermediate 10 in good yield (95%). Chlorination of 10 at C-2 provided 11 , with subsequent β-elimination of HCl in the presence of 1,8-diazabicyclo-[5.4.0]undec-7-ene (DBU), resulting in the formation of the novel C-3-substituted 2,3-unsaturated derivative 12 . The side chain at C-3 could be efficiently extended using an olefin cross-metathesis reaction [12] . Accordingly, reaction of allyl derivative 12 with 4-methylstyrene in the presence of Grubbs' catalyst (second generation) [16] produced the 3-( p -tolyl)allyl derivative 13 in 69% isolated yield (corrected to 77% based on recovered 12 ). We observed that the cross-metathesis reaction was stereoselective and provided the thermodynamically more stable ( E )-isomer. This was confirmed by a 1 H NMR coupling constant ( J 1,2 ) for the trans -olefinic hydrogens of 15.9 Hz. Exposure of 12 and 13 to standard base-catalysed deprotection conditions gave the target 3-allyl-Neu5Ac2en ( 5 ) in a 51% yield (60% yield based on recovered 12 ), and 3-(p-tolyl)allyl-Neu5Ac2en ( 6 ) in a 94% yield, following isolation and purification. Our initial biological evaluation of 5 and 6 against wild-type influenza virus sialidases confirmed that both compounds were selective inhibitors of group-1 sialidases ( Table 1 ). Plaque reduction assay and EC 50 determinations confirmed that 6 selectively inhibited the growth of wild-type N1-containing viruses compared with a wild-type N2-containing virus ( Supplementary Fig. S1 and Supplementary Table S1 ). Importantly, our data revealed that the 2009 pandemic H1N1 virus and N1 sialidase are as sensitive to these C-3 functionalized sialic acid derivatives as the other evaluated group-1 viruses and sialidases. This observation contrasts a very recent report [7] , in which the conclusion reached was that this particular group-1 sialidase lacks a 150-cavity. Therefore, we propose that the 2009 pandemic H1N1 sialidase does have an accessible 150-cavity that is exposed to some extent upon the binding of an appropriate inhibitor such as 5 or 6 . Oseltamivir ( 2 ) resistance among influenza A/H1N1 viruses has rapidly emerged over the previous two influenza seasons [17] . The observation [8] , [17] of significant resistance development to oseltamivir ( 2 ) and apparent reduced [18] sensitivity to zanamivir ( 1 ) led us to investigate the affinity of these novel sialic acid derivatives for three influenza virus sialidases that contain well-characterized key mutations. Each of these sialidases contained one of the following mutations (N2 numbering), H274Y (H275Y in N1 numbering), N294S, or Q136K, which influence the efficacy of the sialidase-targeting drugs. Our data ( Table 1 ) suggest that N1 with an H274Y mutation, which significantly reduces OC ( 3 ) sensitivity [8] , [17] , remains sensitive to 5 and 6 . The level of inhibition for these compounds follows the same apparent trend (approximately a factor of 2 poorer affinity compared with wild-type enzyme) that is observed for both zanamivir ( 1 ) and Neu5Ac2en ( 4 ). The N294S mutation reduces sensitivity to 5 and 6 by approximately the same factor (~3.5) determined for 1 and 4 . Strikingly, the Q136K mutation, that reduces sensitivity to zanamivir ( 1 ) and to a lesser extent 4 , significantly increases sensitivity to the novel sialic acid derivatives 5 and 6 . This improvement in sensitivity may be the result of an increase in hydrophobicity, contributed by the lysine side chain, of the active site region that consequently better accommodates the lipophilic moiety at C-3 of 5 and 6 . These data taken together suggest that a C-3-modified sialic acid derivative, such as 6 , may provide a valuable lead compound for next generation anti-influenza drug discovery. Moreover, the introduction of the additional hydrophobic character may provide opportunity for these compounds, unlike zanamivir ( 1 ), to be developed as orally bioavailable drugs. To provide direct proof of the binding mode of 5 and 6 with a group-1 sialidase, the compounds were soaked into preformed crystals of N8 sialidase [A/duck/Ukraine/1/63 (H3N8)], in which the 150-loop is in the open conformation [5] . The N8– 5 ( Fig. 3a and b , Supplementary Fig. S2 and Supplementary Movie 1 ) and N8– 6 ( Fig. 4a and b , Supplementary Fig. S3 , and Supplementary Movie 2 ) complexes obtained after a 60-min soak show that both 5 and 6 are positioned in the active site as anticipated. In both complexes, the dihydropyran ring, the C-6 glycerol side chain (showing a bidentate interaction between the C-8 and C-9 hydroxyl groups and Glu-276), and the C-4 hydroxyl and C-5 acetamido groups are oriented essentially as seen with Neu5Ac2en ( 4 ) (PDB:2htr) [5] . The C-3 allyl and ( p -tolyl)allyl group of 5 and 6 , respectively, extend into the 150-cavity, as predicted, locking the 150-loop open. Under similar soaking conditions, the N8– 4 complex ( Fig. 4c ) has the 150-loop in a closed conformation [5] . An interesting difference observed in the N8– 5 complex ( Fig. 3 ), compared with the apo structure or the open 150-loop complex with 3 (ref. 5 ), is the position of Arg-118, one of the three arginine residues that normally complexes the Neu5Ac2en carboxylate group. In the N8– 5 complex, Arg-118 is oriented away from the position seen in the other two open 150-loop structures and as a consequence no longer forms a hydrogen bond with the carboxylate group of 5 ( Fig. 5 ). This observation suggests that there is more flexibility in this region of the active site than previously thought and may provide additional direction in future influenza virus sialidase inhibitor development. In a previous molecular modelling study [19] , the notion of flexibility in this region of the active site was predicted. In another study [20] , the triarginyl cluster interaction with the sialic acid carboxylate group has been calculated to contribute ~50% of the overall binding energy and so represents one of the strongest influences on substrate binding to the sialidase active site. The loss of interaction with Arg-118 could be expected to contribute to the in vitro sialidase inhibition observed for 5 in comparison with inhibitors that have interaction with all three residues of the triarginyl cluster. 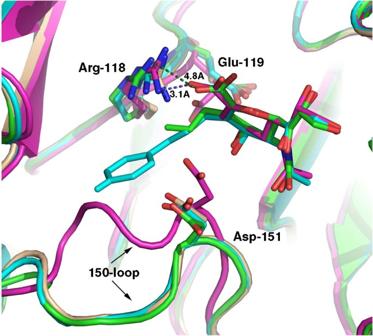Figure 5: Superimposition of N8 structures. Superimposition of the open 150-loop of N8–6(cyan) and N8–5(green),apo-N8 (pale orange; 2ht5) complexes, and the closed 150-loop of N8–4(magenta; 2htr). Figure 5: Superimposition of N8 structures. Superimposition of the open 150-loop of N8– 6 (cyan) and N8– 5 (green), apo -N8 (pale orange; 2ht5) complexes, and the closed 150-loop of N8– 4 (magenta; 2htr). Full size image Although movement of Arg-118 was observed in the N8– 5 complex ( Figs 3 and 5 ), compared with the apo structure or the open 150-loop complex with 3 (ref. 5 ), the N8– 6 complex ( Figs 4 and 5 ) clearly shows that 6 binds in a manner that does not induce any significant reorientation of active site amino-acid residues. The 150-loop structure, the triarginyl cluster that forms a hydrogen bond with the carboxylate group of 6 and other key amino acids are all in a similar orientation [5] to that seen in the apo open 150-loop structure (2ht5) ( Fig. 5 ). Interestingly, the amino-acid residue Glu-119 in the apo form and in both the N8– 5 and N8– 6 complexes has a very similar orientation, and is quite distinct from the closed loop form, as observed in the N8– 4 complex ( Fig. 5 ). Clearly, a reorientation of this residue occurs as the active site closes around inhibitor 4 . The fact that both the parent inhibitor 4 and 6 are micromolar inhibitors suggests that the loss of interactions between the C-4 hydroxyl group of 4 and active site residue Glu-119 of the closed 150-loop form [5] is almost completely compensated for by new hydrophobic interactions between the aromatic moiety at C-3 in 6 and the 150-cavity ( Fig. 6 ). Compound 6 provides a lead scaffold that, guided by structural analysis, can be further modified at the C-3 functionality itself or the C-4 position, as was the case for zanamivir. 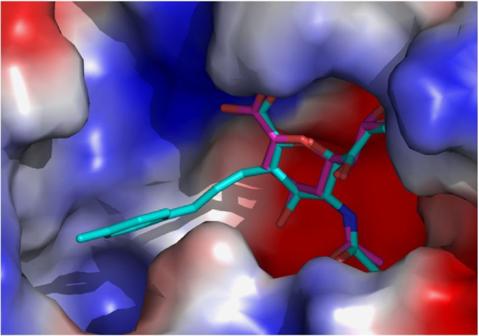Figure 6: Electrostatic potential map of the N8–6complex. N8–6complex showing electrostatic potential on the protein surface (red, negative; blue, positive; and white, neutral/hydrophobic). Neu5Ac2en (4), in magenta, is superimposed on6. As can be seen in Figure 6, the open cavity has significant positive charge character and provides scope for introduction of negatively charged substituents. Such modifications offer considerable opportunity for the development of potent influenza virus sialidase inhibitors. Figure 6: Electrostatic potential map of the N8– 6 complex. N8– 6 complex showing electrostatic potential on the protein surface (red, negative; blue, positive; and white, neutral/hydrophobic). Neu5Ac2en ( 4 ), in magenta, is superimposed on 6 . Full size image In conclusion, we have demonstrated that it is possible, using appropriately substituted Neu5Ac2en derivatives, to lock open the flexible 150-loop of influenza A virus group-1 sialidases. Moreover, these derivatives demonstrate selectivity for an influenza A virus group-1 sialidase compared with a group-2 sialidase and the capacity to inhibit oseltamivir-resistant influenza virus sialidases. Further studies using the C-3-substituted Neu5Ac2en template may help to determine whether group-2 sialidases also possess, as suggested by molecular dynamics simulations [19] , [21] , some plasticity or flexibility in this area of the protein. Finally, the most recent and the most devastating pandemic influenza A viruses, swine origin H1N1 and the 1918 H1N1 respectively, both contain a group-1 sialidase. This study may provide and inform new direction in the discovery of novel influenza virus sialidase inhibitors as next generation, first-line-of-defence, anti-influenza drugs to specifically tackle such viruses. Molecular modelling Superimposition of the influenza A virus sialidase apo -N8 structure (2ht5) and the N8– 4 structure (2htr) using DeepView (Swiss-PDBViewer) [22] was visually inspected in Astex Viewer [23] . Several Neu5Ac2en ( 4 ) derivatives substituted at the C-3 position, including 5 and 6 , were then built in InsightII [24] and docked using AutoDock 3.0.5 (ref. 25 ) into the active site of the apo -N8 structure (2ht5). Specifically, the protein was prepared in the standard manner using AutoDock Tools (version 1.4.5) (ref. 26 ) and a grid of 70 Å×60 Å×60 Å was constructed with a spacing of 0.375 points per Å, centred around the active site. The following parameters were used in the AutoDocking calculations: ga_pop_size=250, ga_num_evals=20,000,000, and 250 docking conformations were generated. The results were processed using the utilities provided with AutoDock [25] and visualized using AstexViewer [23] . AutoDock has been successfully used to predict the binding pose and energy of interaction of known inhibitors in the influenza virus sialidase active site and confirms that AutoDock is able to reproduce experimentally determined binding modes with a high degree of accuracy [27] . Synthesis of sialic acid derivatives The sialic acid derivatives 5 and 6 were prepared according to Figure 2 , using protocols described in the Supplementary Information . 1 H NMR spectra for the key compounds are provided ( Supplementary Figs S4 , S5 , S6 and S7 ). Viruses Influenza virus A/Hong Kong/156/97 (H5N1) and influenza virus A/California/07/2009 (H1N1 pdm) were kindly provided by Alan Hay (NIMR) and by Nancy Cox (Centers for Disease Control), respectively. The influenza viruses A/Paris/0497/2007 (H1N1), A/Paris/2590/2009 (H1N1 pdm) and A/Paris/908/97 (H3N2) were isolated by the National Influenza Center (Northern France) at the Institut Pasteur in Paris (France). Sialidase inhibition assay The sequence encoding the sialidase was amplified from viral RNA by reverse transcriptionPCR, and cloned into the pCI vector (Invitrogen), using standard procedures. Two independent clones were selected for the neuraminidase of each of the three wild-type viruses included in the study. The H274Y, N294S and Q136K mutations were each introduced into a plasmidic clone encoding the N1 of A/Hong Kong/156/97 or A/Paris/2590/2009, using a QuickChange site-directed mutagenesis kit (Stratagene). All constructs were verified by sequencing using a Big Dye terminator sequencing kit and an automated sequencer (Perkin Elmer). Sialidase inhibition assays were carried out on MES-β-dodecyl- d -maltoside cell extracts prepared from 293T cells transiently expressing the viral enzyme, as previously described [13] . Sialidase enzymatic activity was measured using the fluorogenic substrate 2-α-(4-methylumbelliferyl)- d - N -acetylneuraminic acid (Sigma), according to the method of Potier et al . [28] Final concentration of the substrate ranged from 5 to 100 μM. Fluorescence was monitored every 45 s for 20 to 30 min at 37 °C, using a Xenius spectrofluorometer (SAFAS) with excitation and emission wavelengths of 330 and 450 nm, respectively. To measure the inhibitory effect of compounds, cells were preincubated for 30 min at 37 °C in the presence of variable concentrations of the compounds (0.01–10 nM for zanamivir ( 1 ), or 25 nM to 2 μM when tested on the Q136K mutant N1; 0.1–100 μM for Neu5Ac2en ( 4 ); 6.125–800 μM for 5 ; 1–400 μM for 6 ), and the substrate was added at a final concentration of 20 μM. Measurements are the mean of 2–8 experimentally determined values. The kinetic parameters V max , K m and K i were calculated by fitting the data to the appropriate Michaelis Menten equations, using the Levenberg–Marquardt algorithm as provided in the commercially available KaleidaGraph software package (Synergy Software). Cell-based virus inhibition assay The plaque phenotype of the indicated viruses was assayed on MDCK-SIAT cells [29] in the presence of serial dilutions of zanamivir ( 1 , 0.1 nM to 10 μM), Neu5Ac2en ( 4 , 10 nM to 1 mM), 5 (500 nM to 5 mM) or 6 (10 nM to 1 mM), using a plaque assay protocol adapted from a published procedure [30] . Cells were stained with crystal violet after 72 h of incubation at 35 °C. For each inhibitor, the average plaque diameters were plotted against the inhibitor concentrations. The EC 50 was determined graphically as the concentration of inhibitor that induced a 50% reduction in the average plaque diameter. The A/California/07/2009 H1N1 pandemic strain was used in the plaque reduction assay due to its capacity to form larger plaques compared with the corresponding A/Paris/2590/2009 H1N1 pandemic strain. Protein X-ray crystallography N8 sialidase from A/Duck/Ukraine/1/63 (H3N8) was prepared from virus grown in hens' eggs. Sialidase was released from the viruses by bromelain digestion, and further purified, as previously described [5] . N8 sialidase crystals were grown by vapour diffusion in hanging drops consisting of 2 μl of reservoir solution (0.1 M imidazole, pH 8.0 and 35% (±)-2-methyl-2,4-pentanediol (MPD)) and 2 μl of concentrated protein solution (10 mg ml −1 in 10 mM TrisHCl, pH 8.0). A crystal of N8 sialidase was soaked in 1 mM 5 or 6 for 60 min. Data were collected on an in-house rotating anode (RA Micro7 HFM) and a Saturn944 CCD at 100 K and processed with d*Trek [31] . Standard refinement was carried out with a combination of Refmac [32] and PHENIX [33] , together with manual model building with O [34] or Coot [35] . Statistical support for the N8– 5 and N8– 6 structures is presented in Supplementary Table S2 . Structural data have been deposited with the Protein Data Bank with accession codes 3O9J (N8– 5 ) and 3O9K (N8– 6 ). How to cite this article: Rudrawar, S. et al . Novel sialic acid derivatives lock open the 150-loop of an influenza A virus group-1 sialidase. Nat. Commun. 1:113 doi: 10.1038/ncomms1114 (2010).